Propagation style controls lava–snow interactions Understanding interactions between volcanic eruptions and the cryosphere (a.k.a. glaciovolcanism) is important for climate reconstructions as well as for hazard mitigation at ice-clad volcanoes. Here we present unique field observations of interactions between snowpack and advancing basaltic lava flows during the 2012–13 eruption at Tolbachik volcano, Kamchatka, Russia. Our observations show that lava–snow heat transfer is slow, and that styles of lava propagation control snowpack responses. ′A′a and sheet lava flows advance in a rolling caterpillar-track motion on top of the rigid, snowpack substrate with minor lava–snow interaction. In contrast, pahoehoe lava propagates by inflation of lobes beneath/inside the snowpack, producing rigorous lava–snow interaction via meltwater percolation down into the incandescent lava causing production of voluminous steam, rapid surface cooling and thermal shock fragmentation. The textures produced by pahoehoe–snowpack interactions are distinctive and, where observed at other sites, can be used to infer syn-eruption seasonality and climatic conditions. The 2012–13 eruption at Tolbachik volcano, which is located in the central part of the Kamchatka Peninsula ( Fig. 1 ), was characterised by a Hawaiian–Strombolian style eruption that produced ~0.7 km 3 of lava flows extending up to 17 km from the vents and covering 40 km 2 along the volcano’s southern flank [1] . The estimated discharge rate of lava, based on visual estimates and aerial coverage, gradually decreased from ~400–10 m 3 s −1 over the course of the 9-month long eruption [2] . The eruption produced high-alumina basaltic lava that is sparsely plagioclase porphyritic and is similar in composition to the material erupted from the southern fissure during the previous 1975–76 flank eruption at Tolbachik [3] . 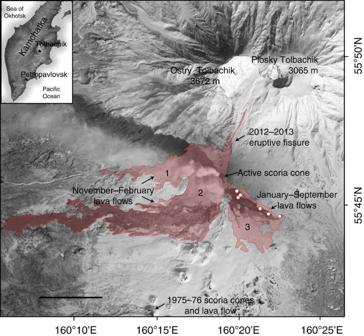Figure 1: Generalised final areal distribution of the 2012–13 Tolbachik lava flow field. Eruption occurred on the southern flank of Tolbachik volcano (lavas shown in translucent pink are superimposed over a NASA EO-1 ALI satellite image taken on 5 April 2013; multiple kipukas are not shown). White eruptive cloud rising above the active scoria cone (the Naboko vent) is drifting towards the northwest. The relative ages of the lava flows can be distinguished by the shades of grey: light-grey—the older flows partly covered by snow; and dark grey—the youngest flows. The merged edifices of Ostry and Plosky Tolbachik volcanoes are in the upper right corner of the image. The summit caldera of Plosky Tolbachik subsided substantially during the 1975–76 fissure eruption. The major branches of the 2012–13 lava flows are identified by numbers: 1—Vodopadnoye field; 2—Leningradskoye field; and 3—Toludskoye field. The Toludskoye lava field was actively growing through the snowpack during the course of this study (observation locations are indicated by circles). The scale bar (lower left) is 4 km in length. The inset shows the location of Tolbachik volcano on the Kamchatka Peninsula. EO-1 image is courtesy of NASA’s Earth Observing One (EO-1) satellite managed by the Goddard Space Flight Center (http://eo1.gsfc.nasa.gov). Figure 1: Generalised final areal distribution of the 2012–13 Tolbachik lava flow field. Eruption occurred on the southern flank of Tolbachik volcano (lavas shown in translucent pink are superimposed over a NASA EO-1 ALI satellite image taken on 5 April 2013; multiple kipukas are not shown). White eruptive cloud rising above the active scoria cone (the Naboko vent) is drifting towards the northwest. The relative ages of the lava flows can be distinguished by the shades of grey: light-grey—the older flows partly covered by snow; and dark grey—the youngest flows. The merged edifices of Ostry and Plosky Tolbachik volcanoes are in the upper right corner of the image. The summit caldera of Plosky Tolbachik subsided substantially during the 1975–76 fissure eruption. The major branches of the 2012–13 lava flows are identified by numbers: 1—Vodopadnoye field; 2—Leningradskoye field; and 3—Toludskoye field. The Toludskoye lava field was actively growing through the snowpack during the course of this study (observation locations are indicated by circles). The scale bar (lower left) is 4 km in length. The inset shows the location of Tolbachik volcano on the Kamchatka Peninsula. EO-1 image is courtesy of NASA’s Earth Observing One (EO-1) satellite managed by the Goddard Space Flight Center ( http://eo1.gsfc.nasa.gov ). Full size image The purpose of this study was to document the interaction of active lava flows on the south flank of Tolbachik volcano ( Fig. 1 ) with the snowpack during the winter of 2013. Although previous workers have made some qualitative observations of ′a′a lava–snowpack interactions [4] , [5] , the goals of this study were to make quantitative measurements of temperatures of lava and associated meltwater, rates of lava advance and snowpack melting and textures produced at the lava–snow interface. Our results show that, contrary to intuition, direct melting of the snowpack by lava flows is slow because of the relatively slow thermal diffusivity of low-density snowpack. Although floods of heated meltwater were observed, they had short durations (tens of minutes) and small volumes. Relatively rapid moving sheets of lava produced few immediately visible signs of interaction with the snow substrate. More slowly moving ′a′a lavas also produced only minor visible steam, mainly where large incandescent blocks from the advancing front rolled onto the snow surface. The slowest advancing lavas were pahoehoe that moved beneath and within the snowpack; these flows produced the most visible steam and have textures that would likely be recognizable if found in ancient deposits, making them candidate paleoclimate proxies for documenting eruptions in snow-dominated environments. Field measurements Our field measurements were made in March—April 2013 along the eastern edge of the actively growing lava field that extended to the east from the main vent (Toludskoye Lava Field [3] ; Fig. 1 ). This area has a ‘rise-and-flat’ topography with maximum gradients <10° on rises. Winter snowpack during the course of the eruption varied in thickness from 0 to 2 m across most of the area, with local thicknesses up to 4 m; it increased episodically during the first 4 months of the eruption (December–March) while air temperatures were below freezing. The density of wind-packed snow was ~400 kg m −3 based on field measurements, implying a porosity of ~50% (ref. 6 ). Propagation of lava flows was documented using time-lapse and conventional video cameras, and temperatures of lava and meltwater were measured using forward looking infrared cameras (FLIR) and type-K thermocouples. Three observation pits up to 3 m deep were dug in the snow in front of advancing lava flows to observe interactions between the lavas, meltwater and snowpack. Two distinct endmember styles of lava flow-front advance were observed during the eruption: (1) tractor-tread (′a′a and sheet flows); and (2) ‘inflation’ (pahoehoe). Lava flow characteristics ′A′a flows were dominant and formed lava tongues hundreds to thousands of metres long, tens of metres wide and with thicknesses of 2–5 m. They were characterised by a rolling, tractor-tread motion, with a friable layer of clinkery autobreccia composed of 0.1–1 m-sized clasts transported on the top of a moving molten lava core ( Fig. 2a ). In the front of the advancing flow, the autobreccia continuously rolled off the flow upper surface and then was overridden by the core of the flow to produce the basal breccia. Temperatures of the incandescent lava core were between 1,253 K (980 °C; FLIR) and 1,328 K (1,055 °C; thermocouple). Surface temperatures of the autobreccia blocks measured with FLIR camera were up to 1,173 K (900 °C). Rates of advance for ′a′a flows were on the order of 0.02 m s −1 . 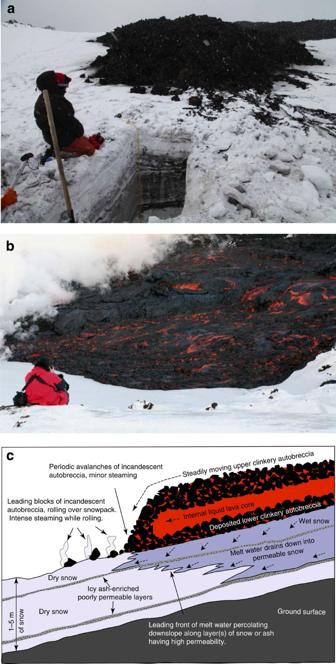Figure 2: Lava flows advancing in tractor-tread style over thick snowpack with little obvious effect. (a) Front of ′a′a lava 2 m thick slowly advancing towards observation pit in the snowpack. Person for scale. (b) Front of a sheet flow 0.5–1 m thick quickly advancing over an area of snowpack 1–4 m deep. Person for scale. (c) Schematic sketch showing a cross-sectional view along the front of an ′a′a flow advancing over thick snowpack. Figure 2: Lava flows advancing in tractor-tread style over thick snowpack with little obvious effect. ( a ) Front of ′a′a lava 2 m thick slowly advancing towards observation pit in the snowpack. Person for scale. ( b ) Front of a sheet flow 0.5–1 m thick quickly advancing over an area of snowpack 1–4 m deep. Person for scale. ( c ) Schematic sketch showing a cross-sectional view along the front of an ′a′a flow advancing over thick snowpack. Full size image Rare, short-lived (hours) sheet flows of lower viscosity lava were also emplaced with a similar style ( Fig. 2b ). The flows were broad (up to 100 m) but thin (<0.5–1 m), and propagated with velocities up to 1–2 m s −1 . The flows had a smooth, elastic, thin outer ‘skin’ that rolled like a tractor tread without breaking into pieces; thus they lacked basal autobreccias. The sheet flows are formed when active lava channels become temporarily obstructed, causing lava to overflow the channel margins and travel across snow-covered slopes. The second endmember emplacement style was observed for pahoehoe flows ( Fig. 3a ), which propagated by sequential slow extrusion and inflation of multiple, individual smooth-surfaced bulbous lava lobes. Each lobe inflated to maximum dimensions of ~1 m before fracturing to produce a new lobe, commonly growing in direction oblique/perpendicular to the parental lobe. Subsequently the whole system of interlaced and interconnected lobes continued to inflate slowly. Temperatures inside of the incandescent lava lobes were up to 1,353 K (1,080 °C; thermocouples), and temperatures of the lava lobe surfaces were up to 1,273 K (1,000 °C; FLIR). Advance rates for pahoehoe lava flows were in the order of 0.008 m s −1 . 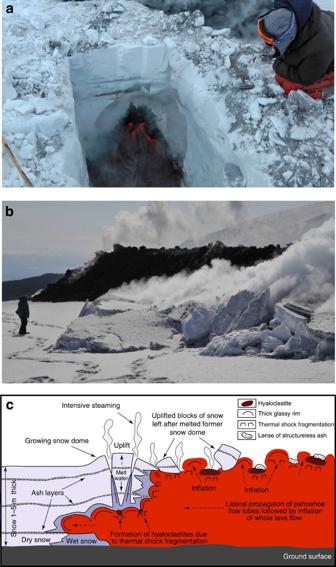Figure 3: Lava flows advancing via inflation beneath/inside thick snow pack. (a) Front of pahoehoe lava advancing beneath the snowpack; base of the flow is ~2 m below the snow surface, leading part of the flow ~1 m below the snow surface and the leading lobe is entering lower part of observation pit. Pit is ~1 m wide. (b) Growing snow dome with steam emanating from hidden contact between melting snow and inflating subsnow pahoehoe flow; in the background ′a′a lava 4 m thick advancing over snow. Person for scale. (c) Schematic sketch showing cross-sectional view along the front of pahoehoe flow advancing through the snow. Figure 3: Lava flows advancing via inflation beneath/inside thick snow pack. ( a ) Front of pahoehoe lava advancing beneath the snowpack; base of the flow is ~2 m below the snow surface, leading part of the flow ~1 m below the snow surface and the leading lobe is entering lower part of observation pit. Pit is ~1 m wide. ( b ) Growing snow dome with steam emanating from hidden contact between melting snow and inflating subsnow pahoehoe flow; in the background ′a′a lava 4 m thick advancing over snow. Person for scale. ( c ) Schematic sketch showing cross-sectional view along the front of pahoehoe flow advancing through the snow. Full size image Lava–snowpack interactions In areas having thin (<0.5 m) snowpack and/or featuring slowly advancing lava (<0.008 m s −1 ), both endmember types of lava flows produced notable melting of snowpack. Locally, where the lava flows approached the vertical walls of the edge of the snowpack, steam and meltwater were observed. The meltwater either saturated snow in front of the lava or formed continuous short streams that refroze after travelling distances of tens to hundreds of metres after emerging from the base of lava flow-fronts. Where observed, the visually estimated discharge rate of meltwater was generally small (~1–5 l s −1 ); the highest rates (~30 l s −1 ) were estimated from small streams emanating from beneath the front of ′a′a lava flows. Meltwater temperatures varied but within 5 m of the lava flow-fronts were as high as 333 K (60 °C). In areas where lava flows advanced over snow thicker than ~0.5 m, the ′a′a/sheet lava flows advanced over the snow surface, and produced few obvious melting such as visible steam or meltwater. Locally, small steam plumes were visible for a few seconds when incandescent blocks tumbled directly onto the snowpack, which acted as a rigid substrate ( Fig. 2c ). At most locations even 2 m of snow had enough strength to temporarily support advancing ′a′a lava flows >3 m thick, although propagation of fractures within the snowpack beneath flows was frequently audible. Observation pits dug into the snow in front of the flows showed that almost no continuous melting was occurring directly under the fronts of advancing ′a′a flows ( Fig. 2b ), although in some cases ephemeral lenses of meltwater migrated through the lower sections of the snowpack several metres ahead of advancing lava flows. Repeat visits to the same areas showed that ′a′a flows completely melted through snow cover in less than 24 h. Locally, where snowpack was <1 m, and presumably the meltwater volume exceeded the pore space in the snowpack, small, short-lived meltwater floods emanated from beneath the front of lava flows. The water discharge events were generally of short duration, lasting several minutes. In a few instances meltwater-saturated snow collapsed beneath thickening ′a′a flows. In contrast, pahoehoe lava flows advanced beneath or within the thick snowpack. Snow acted as a brittle medium through which lava advanced by a combination of melting/evaporation and brittle deformation ( Fig. 3c ). Observations pits in front of pahoehoe flows showed that the snow remained rigid and fractured brittlely as the lava advanced through it, with limited observed melting that only occurred within the first few cm of snow at the contact with growing lobes. In some instances, blocks of snow were pushed in front of the advancing lava flows creating thrust fault-bounded snow blocks. Arcuate, subvertical cracks in the snow formed where lavas burrowed into thicker snow banks (>3 m), and in one instance a ‘dike’ of lava was observed intruding into a fracture between two snow blocks. Leading lava lobes deposited beneath/inside snowpack subsequently slowly inflated, locally producing doming of the overlying snow ( Fig. 3b ), which grew at rates of cm per minute until the snow fractured into large blocks. Meltwater from the growing snow dome percolated down into the underlying hot lava, chilling the lava and producing voluminous steam clouds. As a result, upper surfaces of these flows had thick glassy rims (>2 × 10 −2 m), and locally were intensively fractured by thermal stress, producing localised zones of vitric fragments (hyaloclastite). Within several hours of deposition of the pahoehoe lava flows, snow domes gradually melted, leaving behind on the lava surface scattered snow blocks and structureless lenses of older tephra that had been originally intercalated with the snowpack. Observations of sheet lavas moving across the uncovered snowpack or pahoehoe flows inflating inside snowpack have never been reported before, and even observations of ′a′a–snow interactions are limited [4] , [5] . During the 1947 Hekla and the 2010 Fimmvörðuhals eruptions in Iceland, ′a′a flows were observed moving across snow with little obvious effect on the snow [4] , [5] . At Hekla it was speculated that the basal lava breccia insulated the snow from the lava [4] , and at Fimmvörðuhals an insulating effect was attributed to tephra that covered the snowpack [5] . The new observations from Tolbachik clearly show that presence of such extra insulators is not required for the lava to flow on top of the snow: when rapidly advancing lava comes into direct contact with snow, the lava immediately developed a thin, chilled crust that provides significant thermal insulation. Additionally, given estimated snow densities at Tolbachik, the thermal diffusivity of the snowpack would be ~0.5 × 10 −6 m 2 s −1 , which is of the same magnitude as that for the lava [6] . The relatively high porosity estimated for the Tolbachik snowpack means that meltwater, which if present at the lava–snow boundary would significantly increase rates of heat transfer, rapidly drained down into the snowpack and away from the lava–snow interface. This explains why only small, localised floods and small rare phreatomagmatic explosions were witnessed during the 2012–2013 Tolbachik eruption. Past workers have used two different approaches to quantify rates of heat transfer from lava to snow/ice [5] , [7] . The first approach is theoretical and assumes heat transfer into ice either below or above the lava solely by conduction [7] . While this approach makes several simplifying assumptions (for example, fixed boundary layers, no water or steam present at the boundary, instantaneous emplacement), it gives order of magnitude estimates of ice melting rates for lava flows of different thicknesses (1, 3, 10 and 30 m) and predicts heat fluxes. Modelled instantaneous rates of melting vary from a high of 8.5 × 10 −5 m s −1 for a 1-m thick lava flow within the first 10 min of lava–ice contact, to 5.9 × 10 −6 m s −1 after 1.5 days. Based on the reported instantaneous rates of melting, an estimate of the integrated thickness of snow melted in 1 day is 3.7 m for a 1-m thick lava flow, and 2.4 m for a 3-m thick lava flow ( Fig. 4 ). 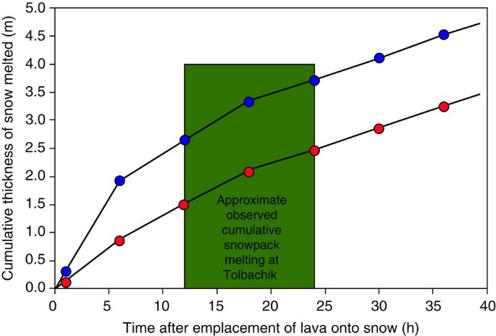Figure 4: Estimates of cumulative ice melting via conduction as a function time. Cumulate curves for 1 m thick (blue circles) and 3 m thick (red circles) lavas are based on integrated, linear approximations of instantaneous melting rates7. Shaded green box shows estimated cumulative thicknesses of snow melted and time-scales of melting beneath Tolbachik lava flows for comparison. Figure 4: Estimates of cumulative ice melting via conduction as a function time. Cumulate curves for 1 m thick (blue circles) and 3 m thick (red circles) lavas are based on integrated, linear approximations of instantaneous melting rates [7] . Shaded green box shows estimated cumulative thicknesses of snow melted and time-scales of melting beneath Tolbachik lava flows for comparison. Full size image The second approach is based on observations of melting rates from the 2010 Fimmvorduhals eruption [5] and large-scale experiments [8] . The heat flux from the base of the lava flow can be constrained using the observed overall rate of melting, given the depth of snow melted (Δ x ) as a function of time ( t ), the density of the snow ( ρ s ) and the latent heat of fusion for ice [6] ( L i =3.35 × 10 5 J K −1 ) by: Given the observations from this study, where Δ x varied from 1 to 3 m over time periods of 12–24 h for a measured ρ s of 400 kg m −3 , the implied heat fluxes from the base of lava flows were in the range of 155–9,300 W m −2 , which are consistent with the previous observational and theoretical estimates [5] , [7] , [8] . Past workers concluded that the potential for lahar generation from lava–snow/ice interaction is relatively minor compared with that of pyroclastic eruptions, although several examples of lava-generated lahars are known [9] . Our observations also show that the majority of the slow moving lava flows at Tolbachik were emplaced at rates that were too low (<0.3 m s −1 ) to allow for the rapid production of large meltwater volumes. For example, the slow moving ′a′a flows typical of Tolbachik (~20 m wide, advancing at 0.01 m s −1 ) could melt ~1,200 m 2 of snowpack in 1 h. Assuming a snowpack depth of 2 m, the resulting meltwater production rate would be ~0.1 m 3 s −1 if all of the snow melted within 1 h. For a stream channel with a cross-sectional area of 1 by 1 m, this would produce a flow 0.1 m in height moving at a velocity of 1 m s −1 . Thus, in the absence of a mechanism to impound meltwater over long time periods (that is, several days), slow moving lava flows emplaced onto snowpack seem unlikely to produce significant flooding hazards. It has also been suggested that lava mainly interacts vigorously with snow/ice/frozen ground (with generation of phreatomagmatic explosions and lahars), where rapid intermixing of lava with the frozen substrate is facilitated by gravity-drive collapse of lava flows on steeps slopes [10] . These new observations also have important implications in studies of interactions between volcanoes and climate [11] , [12] , [13] . At present, more than 500 active volcanoes on Earth (~one-third) are estimated to have at least seasonal snow/ice cover based on their elevations, latitudes and reported locations with respect to the existing glaciers [14] , [15] . Obviously more volcanoes were snow-clad during past glaciations when the global extent of snow- and ice-cover was higher than today. Thus it is reasonable to assume that effusive lava–snow interactions were more frequent during waxing and waning of glacial stades, where the resulting deposits can be identified they will be valuable as local paloeclimate/seasonality proxies (for example, recording the presence of snow). Recognition of such deposits could be used to identify retreating snow-lines during periods of climate warming, to investigate possible connections between eruptions and seasonality, or even document the length of the eruption if lava flow fields contain examples of lava–snow interaction in addition to lava textures indicative of snow-free conditions. Lava–ice interactions have also long been inferred to have occurred on Mars [16] , [17] . Verification of the origins of those deposits is increasingly important as environments where volcanism could have produced hydrothermal fluids are likely targets for exo-life exploration [18] . With increasingly detailed observations from the surface of Mars such as the recognition of purported cooling fractures on surfaces of an exposed lava [19] , it may soon be possible to identify the characteristic deposits produced by lava–snow interactions there and on other solar system bodies as well. This may in turn lead to more accurate and detailed paleoclimate history reconstructions and a better understanding of planetary climate. How to cite this article: Edwards, B. R. et al . Propagation style controls lava-snow interactions. Nat. Commun. 5:5666 doi: 10.1038/ncomms6666 (2014).